Delocalization and dielectric screening of charge transfer states in organic photovoltaic cells Charge transfer (CT) states at a donor–acceptor heterojunction have a key role in the charge photogeneration process of organic solar cells, however, the mechanism by which these states dissociate efficiently into free carriers remains unclear. Here we explore the nature of these states in small molecule–fullerene bulk heterojunction photovoltaics with varying fullerene fraction and find that the CT energy scales with dielectric constant at high fullerene loading but that there is a threshold C 60 crystallite size of ~4 nm below which the spatial extent of these states is reduced. Electroabsorption measurements indicate an increase in CT polarizability when C 60 crystallite size exceeds this threshold, and that this change is correlated with increased charge separation yield supported by CT photoluminescence transients. These results support a model of charge separation via delocalized CT states independent of excess heterojunction offset driving energy and indicate that local fullerene crystallinity is critical to the charge separation process. Charge transfer (CT) states at a donor–acceptor heterojunction (DA HJ) are increasingly recognized as key in determining both the practical and thermodynamic limiting efficiency of organic photovoltaic cells [1] , [2] , [3] , [4] , [5] , [6] . These states result from photoinduced CT at the DA HJ and consist of a Coulombically correlated hole and electron perceived to reside on adjacent (or closely neighbouring) donor and acceptor molecules, respectively. Although the important role of CT states in determining photocurrent generation and open-circuit voltage has been established [7] , [8] , [9] , the means by which they overcome an estimated binding energy ~10 k b T to achieve efficient charge separation at room temperature has been the subject of debate [1] , [2] . The classical Coulomb estimate of relaxed CT-binding energy, E B = q 2 /4π εr CT , depends inversely on dielectric constant, ε , and the length r CT , which reflects some average electron and hole separation indicative of the CT spatial extent [2] . It is unclear, however, what the relevant frequency range of ε ( ω ) is or even how much influence such a macroscopically averaged quantity should have on states existing between adjacent molecules. An alternative perspective has emerged from recent spectroscopic investigations suggesting that, at early times following CT (<1 ps), delocalized CT states can be populated that efficiently sample and decay into free charge carriers before ever localizing in the Coulomb well [3] , [4] . Here, we explore the dependence of CT energy, E CT , on background dielectric constant directly via electroluminescence (EL), photoluminescence (PL) and absorption by varying the blend ratio of small molecule–bulk heterojunction (BHJ) organic solar cells based on the donor N , N ′-bis(1-naphthyl)- N , N ′-diphenyl-1,1′-biphenyl-4,4′-diamine (NPD) and the acceptor C 60 . Consistent with previous observations, we observe a red-shift of E CT with increasing C 60 fraction [10] , [11] , [12] , [13] , [14] , but find that modelling based on the accompanying change in dielectric constant via the solid-state solvation effect (SSSE) [15] can only explain the data at high (>50%) C 60 loading. We find that E CT at low fullerene concentration is higher than expected from the change in dielectric constant and attribute this discrepancy to increased localization of the electron component of the CT state because of a reduction in average C 60 crystallite size below ~4 nm. Using electroabsorption (EA) spectroscopy [16] , we observe a substantial increase in CT state polarizability beyond this threshold crystallite size indicative of increasing delocalization, and find that this leads to rapid decay in the CT PL transient attributed to efficient long-range charge separation. These results point to the importance of local crystallinity in enabling delocalization of at least one component (e − or h + ) of the CT state as well as the need to include multiple donor and acceptor molecules in theoretical modelling to accurately capture extended CT states relevant in the charge separation process. CT energy dependence on dielectric constant BHJ devices were fabricated with active layer composition ranging from 20 to 90% C 60 according to the relative co-deposition ratios 4:1, 2:1, 1:1, 1:4 and 1:9 NPD to C 60 . Capacitance–voltage measurements were subsequently carried out at a frequency of 100 kHz with devices depleted in reverse bias (−2 V) to extract the low frequency relative dielectric constant ( ε static ) of each BHJ layer. These data are plotted in Fig. 1a together with the optical frequency dielectric constants ( ε optical ) fit from spectroscopic ellipsometry at an energy E =1.26 eV near the peak of the CT state emission. There is little difference between ε static and ε optical and both vary approximately linearly with C 60 fraction, consistent with expectations of an effective medium description. 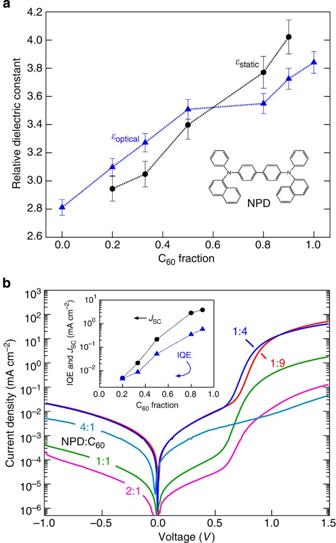Figure 1: Dielectric constant variation. (a) Static (100 kHz) and optical frequency dielectric constants measured as a function of C60volume fraction in the blend. The molecular structure ofN,N′-bis(1-naphthyl)-N,N′-diphenyl-1,1′-biphenyl-4,4′-diamine (NPD) is shown in the inset. Error bars forεopticalreflect standard error in the ellipsometry fits, whereas those forεstaticindicate standard deviations obtained over multiple device measurements. (b) Dark current–voltage characteristics of bulk heterojunction (BHJ) devices with different NPD:C60ratios. Inset: short-circuit currents (Jsc) and internal quantum efficiencies (IQE,λ=450 nm) of the different BHJ devices. Figure 1: Dielectric constant variation. ( a ) Static (100 kHz) and optical frequency dielectric constants measured as a function of C 60 volume fraction in the blend. The molecular structure of N , N ′-bis(1-naphthyl)- N , N ′-diphenyl-1,1′-biphenyl-4,4′-diamine (NPD) is shown in the inset. Error bars for ε optical reflect standard error in the ellipsometry fits, whereas those for ε static indicate standard deviations obtained over multiple device measurements. ( b ) Dark current–voltage characteristics of bulk heterojunction (BHJ) devices with different NPD:C 60 ratios. Inset: short-circuit currents ( J sc ) and internal quantum efficiencies (IQE, λ =450 nm) of the different BHJ devices. Full size image The dark current density–voltage ( J-V ) characteristics of each device are shown in Fig. 1b together with their short-circuit currents ( J sc ) under AM1.5G illumination and internal quantum efficiency (IQE) measured at λ =450 nm (inset). Similar to many polymer/fullerene [11] and evaporated [17] BHJs, we find that overall efficiency is maximized at high C 60 concentration because of a substantial drop in J sc with increasing NPD fraction, which is primarily due to decreasing IQE as opposed to reduced C 60 absorption (NPD absorbs little sunlight with a 3.1-eV optical gap). The functional form of the J-V characteristic is qualitatively maintained with increasing NPD fraction up to 2:1 NPD:C 60 loading, indicating that current is controlled by the same DA HJ generation/recombination processes [9] , albeit with different strengths expected from changing carrier mobilities and recombination rates [18] . 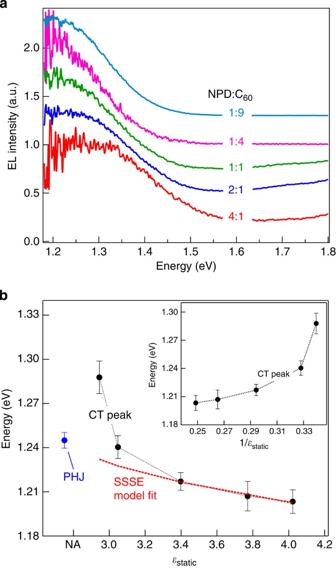Figure 2: Charge transfer emission energy dependence on dielectric constant. (a) Electroluminescence (EL) spectra indicating a shift in charge transfer (CT) emission in cells with varyingN,N′-bis(1-naphthyl)-N,N′-diphenyl-1,1′-biphenyl-4,4′-diamine (NPD):C60ratio. The spectra are normalized and shifted vertically for clarity. (b) EL peak energies extracted from fitting and plotted as a function of static dielectric constant. The red dashed line indicates the prediction of solid-state solvation theory (SSSE) described in the text. The inset shows the same CT peak energies plotted versus inverse dielectric constant. Error bars indicate standard error obtained in the EL peak fitting ofa. NA, not applicable; PHJ, planar heterojunction. Figure 2a shows the EL spectra measured under forward bias at current densities of 75 mA cm −2 , which exhibit a peak assigned to an NPD-C 60 CT state that red-shifts from approximately 1.3 to 1.2 eV with increasing C 60 concentration. This CT state is the sole EL component in the 1:9, 1:4 and planar HJ device spectra, whereas some NPD and C 60 excitonic emission (at peak energies E =2.9 eV and 1.67 eV, respectively; see Supplementary Fig. 1 ) is observed in the 1:1, 2:1 and 4:1 spectra as higher bias (up to 4 V) was needed to achieve a current density with sufficient signal to noise in the CT emission. No measurable change in CT emission energy was observed as a function of bias (see Supplementary Fig. 2 ), indicating that filling within the disorder-induced CT density of states is negligible in these measurements. Figure 2: Charge transfer emission energy dependence on dielectric constant. ( a ) Electroluminescence (EL) spectra indicating a shift in charge transfer (CT) emission in cells with varying N , N ′-bis(1-naphthyl)- N , N ′-diphenyl-1,1′-biphenyl-4,4′-diamine (NPD):C 60 ratio. The spectra are normalized and shifted vertically for clarity. ( b ) EL peak energies extracted from fitting and plotted as a function of static dielectric constant. The red dashed line indicates the prediction of solid-state solvation theory (SSSE) described in the text. The inset shows the same CT peak energies plotted versus inverse dielectric constant. Error bars indicate standard error obtained in the EL peak fitting of a . NA, not applicable; PHJ, planar heterojunction. Full size image The CT red-shift with increasing fullerene concentration has previously been attributed to the accompanying increase in dielectric constant ( c.f. Fig. 1a ) [10] , [11] . To test this hypothesis, the CT peak energies were extracted from Gaussian multipeak fitting and plotted in Fig. 2b against ε static and its inverse (inset). A nearly identical dielectric constant dependence was observed for the CT peak in PL as well (see Supplementary Fig. 3 ). The energy shift can be partially explained via the SSSE, which successfully describes the emission red-shift of other polar excited states with increasing dielectric constant in organic thin films [15] . Here, the energy shift Δ E em =− AΛ static − BxΛ optical accounts for screening by the induced local electric field and involves contributions from both the static and optical frequency dielectric constants according to the local field factors Λ =2( ε −1)/(2 ε +1) and constants A and B that depend on the ground and excited state dipole moments involved in the optical transition. Comparing this relationship to the data of Fig. 2 , we find that it can account for the emission energy shift of the 1:9, 1:4 and 1:1 BHJs, but that it fails at lower C 60 fraction. The SSSE fit indicated in Fig. 2b is not unique because of the similarity between ε static and ε optical (that is, A and B are correlated); however, the key point here is that this description cannot, even in principal, describe the full data range—there is simply more curvature in the emission energy shift than the SSSE model is able to predict. Alternatively, Veldman et al. [11] explained shifts in polymer/fullerene CT emission according to an electrostatic expression for the Gibbs free energy for photoinduced electron transfer, which carries the Coulomb electrostatic scaling Δ E em 1/ εr CT . However, as evident in the inset of Fig. 2b , the emission observed here does not shift linearly with inverse dielectric constant, suggesting that the CT spatial extent (that is, r CT ) may be changing at low C 60 fraction. A change in CT energy is also inferred in absorption through sensitive measurement of the external quantum efficiency (EQE). These data are shown in Fig. 3a and feature an absorption tail below the NPD and C 60 optical gaps (see Supplementary Fig. 4 ) that clearly red-shifts with increasing C 60 concentration. 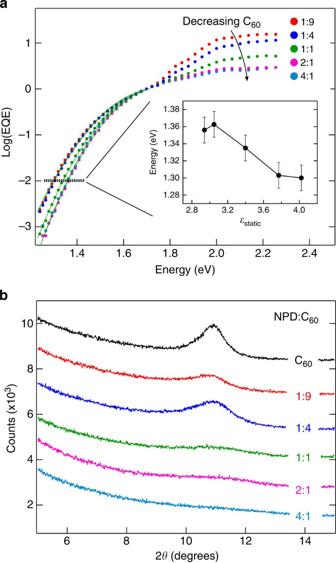Figure 3: Charge transfer state absorption and local fullerene order. (a) External quantum efficiency (EQE) data for devices with varyingN,N′-bis(1-naphthyl)-N,N′-diphenyl-1,1′-biphenyl-4,4′-diamine (NPD):C60ratio, normalized at 1.7 eV for comparison. Green lines indicate fits to Equation 1 in the text and the inset displays the energy shift occurring along the dashed line at constant EQE=10−2. Error bars in the inset reflect the standard deviations estimated from EQE measurements on multiple devices. (b) Glancing incidence X-ray diffraction data for each of the bulk heterojunction films along with a neat C60film. Similar to previous analyses of polymer/fullerene blends [7] , [19] , we assign this feature to absorption from the CT state and find that its low-energy tail can be described by the relationship: Figure 3: Charge transfer state absorption and local fullerene order. ( a ) External quantum efficiency (EQE) data for devices with varying N , N ′-bis(1-naphthyl)- N , N ′-diphenyl-1,1′-biphenyl-4,4′-diamine (NPD):C 60 ratio, normalized at 1.7 eV for comparison. Green lines indicate fits to Equation 1 in the text and the inset displays the energy shift occurring along the dashed line at constant EQE=10 −2 . Error bars in the inset reflect the standard deviations estimated from EQE measurements on multiple devices. ( b ) Glancing incidence X-ray diffraction data for each of the bulk heterojunction films along with a neat C 60 film. Full size image which is characteristic of a transition based on Marcus photoinduced electron transfer [7] , [20] . Here, λ r is the reorganization energy and the constant C 0 includes the transition dipole moment. Fits to this expression (green lines) yield CT absorption maxima with an average of E CT + λ r =1.85 eV, although the imprecision expected in fitting only half of the inverted parabola introduces correlation between the vertex position and broadening parameters that precludes us from establishing a meaningful trend among the different NPD:C 60 blend ratios. Instead, we quantify the shift by plotting the energy change at a constant EQE value identified by the dashed line as shown in the inset [21] . Although it is difficult to distinguish whether this trend is due to a shift or broadening of the CT transition (more insight is obtained from EA below), the ~70 meV overall magnitude of the change is at least qualitatively consistent with that observed in the EL and PL measurements. In addition to dielectric constant, the degree of C 60 crystallinity in the BHJs reduces with decreasing C 60 concentration as evident from glancing incidence X-ray diffraction data shown in Fig. 3b and well-documented in polymer-fullerene systems [13] , [14] , [22] . Application of the Scherrer equation to Gaussian fits of the C 60 reflection at ~11° yields average crystallite sizes of 8.1, 6.5, 5.6, 4.2 and 3.8 nm for the pure C 60 , 1:9, 1:4, 1:1 and 2:1 BHJ films, respectively. No peak could be extracted from either the 4:1 BHJ or neat NPD films as they are highly disordered and most likely amorphous. Based on these observations, we hypothesize that the increase in CT emission energy at low C 60 concentration, also noted by Piersimoni et al. [13] and Muller et al. [14] in polymer-fullerene blends, is due to confinement of the wavefunction as C 60 crystallite size becomes comparable to the natural spatial extent of the CT state (that is, that for large crystallites where CT volume is not influenced by the crystallite boundaries), similar to the manner in which exciton energy increases with decreasing inorganic semiconductor quantum dot size [23] . In this scenario, the electron component of the CT wavefunction in 1:9 and 1:4 BHJs is delocalized over two or three C 60 molecules within a crystallite, whereas the hole remains localized on an adjacent NPD molecule. This estimate is based on the 1.42 nm C 60 FCC lattice spacing, which corresponds to approximately three C 60 molecules in any given dimension for the average 4.2 nm crystallite in the threshold 1:1 BHJ; further reduction in crystallite size increasingly confines the electron and raises the overall energy of the CT state. CT state EA We have examined this possibility further by conducting EA measurements, depleting each cell at −1 V bias and adding a 300-mVrms dither at a frequency of 1 kHz to create a uniform applied field F = F DC + F AC cos(ω t ) throughout the device. The Stark shift in transition energy because of this field is obtained from second-order perturbation theory as ΔE = −Δμ·F −[1/2] Δ F 2 , where Δμ is the difference between ground and excited state dipole moments and Δ is the average change between the ground and excited state polarizability tensors [16] , [24] . Taylor expanding the change in absorption coefficient due to this energy shift as Δ α = α ′Δ E +[ α ″/2](Δ E ) 2 and averaging over randomly oriented molecules/crystallites, we find the first-order (rms) response at the modulation frequency [16] , [24] : The differential transmission is measured with a lock-in amplifier and is related to the change in absorption coefficient, d Δ α =−Δ T / T , where the optical path length d is double the active layer thickness as light is collected in reflection off the Ag cathode. Equation 2 predicts that the EA spectrum will follow the negative first derivative of the absorption coefficient (− α ′) if a polarizability shift dominates, as in the case of, for example, delocalized J-aggregate excitons [25] , whereas it will follow the second derivative ( α ″) if the change in dipole moment is dominant as expected for CT states. 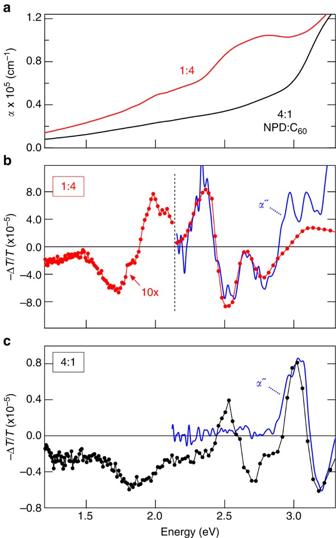Figure 4: Electroabsorption (EA) spectra. (a) Linear absorption coefficients measured for 1:4 and 4:1N,N′-bis(1-naphthyl)-N,N′-diphenyl-1,1′-biphenyl-4,4′-diamine (NPD):C60films. (b) EA spectra collected for the 1:4 device and (c) for the 4:1 device. Blue lines show second derivatives (α'') of the respective absorption coefficients scaled in magnitude to the EA data. Figure 4 shows the EA spectra obtained for the 1:4 and 4:1 devices along with their respective linear absorption coefficients. At energies >2.2 eV, the 1:4 EA spectrum in Fig. 4b is dominated by a second derivative lineshape arising from known CT transitions in bulk C 60 that yield a dipole moment of Δ μ =24 D (refs 24 , 26 ). The 4:1 spectrum in Fig. 4c is correspondingly dominated by the second derivative NPD feature at 3 eV, although the magnitude of the dipole moment Δ μ =5 D is much smaller because of the Frenkel nature of the NPD exciton. The C 60 feature in this case, which is below the derivative resolution of the linear absorption, is blue-shifted relative to the 1:4 BHJ, likely due to a combination of smaller crystallite size and lower dielectric constant. Figure 4: Electroabsorption (EA) spectra. ( a ) Linear absorption coefficients measured for 1:4 and 4:1 N , N ′-bis(1-naphthyl)- N , N ′-diphenyl-1,1′-biphenyl-4,4′-diamine (NPD):C 60 films. ( b ) EA spectra collected for the 1:4 device and ( c ) for the 4:1 device. Blue lines show second derivatives ( α '') of the respective absorption coefficients scaled in magnitude to the EA data. Full size image In both spectra, we observe additional features below 2.2 eV that are not evident in the EA of either pure NPD or C 60 devices (see Supplementary Fig. 5 ). The most evident is located at ~1.85 eV, which corresponds closely with the CT absorption maximum identified through EQE fitting in Fig. 3a . The fact that these devices are depleted and this feature maintains the same modulation frequency dependence (up to the 250 kHz upper limit of the lock-in) as the higher energy excitonic EA is evidence against charge modulated (that is, polaron) absorption and thus we assign the 1.85 eV feature to CT EA. 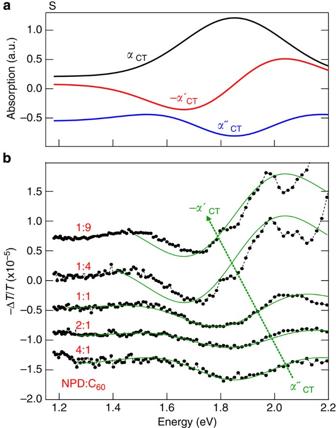Figure 5: Evolution of charge transfer (CT) state electroabsorption. (a) CT absorption lineshape (αCT) along with its first (α'CT) and second (α''CT) derivatives estimated according to Equation 1 of the text and the green line fits inFig. 3a. (b) Low-energy electroabsorption spectra for each NPD:C60BHJ ratio, showing a systematic increase in first derivative lineshape component with increasing C60fraction. BHJ, bulk heterojunction; NPD,N,N′-bis(1-naphthyl)-N,N′-diphenyl-1,1′-biphenyl-4,4′-diamine. Figure 5 provides a closer examination of the CT EA, where we observe a systematic change in moving from a dip in the 4:1 BHJ to a first derivative shape in the 1:9 device. Reproducing the CT absorption lineshape ( α CT ) fit from the EQE in Fig. 5a , we see that the dip corresponds to the second derivative, α ″ CT , expected for a typical CT transition in the 4:1 blend, but that this steadily evolves to include a growing contribution of first derivative lineshape (− α ′ CT ) in the 1:9 blend, indicating a substantial increase in polarizability. This is demonstrated qualitatively by the green lines in Fig. 5b that comprise weighted superpositions of − α ′ CT and α ″ CT , where the contribution from − α ′ CT grows from negligible in the 4:1 to dominant in the 1:9 BHJ. For the sake of transparency, no attempt is made to incorporate the increasing high energy C 60 -related background in the 1:4 and 1:9 mixtures. Figure 5: Evolution of charge transfer (CT) state electroabsorption. ( a ) CT absorption lineshape ( α CT ) along with its first ( α ' CT ) and second ( α '' CT ) derivatives estimated according to Equation 1 of the text and the green line fits in Fig. 3a . ( b ) Low-energy electroabsorption spectra for each NPD:C 60 BHJ ratio, showing a systematic increase in first derivative lineshape component with increasing C 60 fraction. BHJ, bulk heterojunction; NPD, N , N ′-bis(1-naphthyl)- N , N ′-diphenyl-1,1′-biphenyl-4,4′-diamine. Full size image The significant increase in polarizability suggests that the CT state becomes increasingly delocalized and occupies a greater volume at high C 60 loading. This is both intuitively evident and more rigorously from the matrix elements that make up the polarizability, p CT ~ /( E n − E CT ), as these reflect the ease with which neighbouring states, | ψ n , mix with the CT state, | ψ CT (ref. 27 ). Quantitative extraction of the CT dipole moment and its growing polarizability is not possible directly from the linear absorption data in Fig. 4a as first- and second-derivative components of the weak CT absorption cannot be resolved from background noise fluctuations (for example, small differences in reflection and/or scattering). Employing a more sensitive, non-transmission-based absorption technique such as photothermal deflection spectroscopy could resolve this issue. Nevertheless, based on the known slope of α CT according to Equation 1 and its approximate absorption coefficient relative to C 60 from EQE, we estimate μ CT >20 D in the 4:1 blend and CT ~2,600 Å 3 in the 1:4 and 1:9 BHJs, which is roughly three times larger than the polarizability found for the CT-related transitions at 2.4 eV in pure C 60 (ref. 24 ). 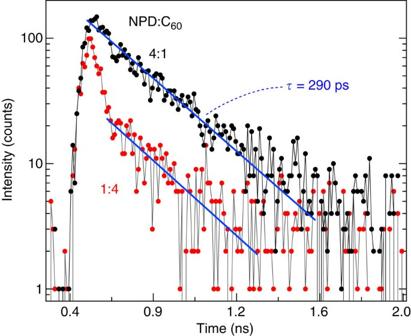Figure 6: Charge transfer (CT) state lifetime. Transient CT photoluminescence in the energy range 1.39–1.45 eV for bulk heterojunctions with high (1:4) and low (4:1) C60fraction. PL transient data of the CT emission shown in Fig 6 indicate that delocalization is accompanied by a significant difference in decay dynamics. Whereas the localized CT state in the 4:1 blend exhibits an approximately monoexponential decay with lifetime τ =290±10 ps, the 1:4 blend displays a rapid initial decay followed by the same lifetime. This rapid initial decay reflects dissociation of delocalized CTs, whereas the low-level τ =290 ps tail is probably due to decay of localized CTs in the fraction of smaller (sub-4 nm) C 60 crystallites within the BHJ ensemble. Figure 6: Charge transfer (CT) state lifetime. Transient CT photoluminescence in the energy range 1.39–1.45 eV for bulk heterojunctions with high (1:4) and low (4:1) C 60 fraction. Full size image Taken together, our observations point to an important role of local fullerene order (and also potentially of the donor in other material systems) beyond a threshold crystallite size of ~4 nm in enabling CT delocalization that is key to efficient long-range charge separation. Moreover, in the presence of sufficiently sized C 60 crystallites, CT delocalization is not dependent on excess driving energy from the initial CT reaction as it is observed here under resonant EA excitation [28] , [29] . The impact of fullerene nanocrystallinity on charge separation has been noted previously, where it was attributed to high local electron mobility within the traditional Onsager framework [11] , [30] as well as to shifts in electron affinity of the fullerene crystallites [31] . In contrast, our results here point to the role of delocalization, analogous to recent findings for organic–inorganic HJs [32] , and are consistent with a growing number of recent reports in which charge separation is driven by accessing band-like CT states that subsequently decay on a sub-50 ps timescale (an upper limit based on the resolution of our PL transient data) into separated, free charge carriers [3] , [4] , [29] , [33] . In summary, these results support a model of delocalized CT state dissociation and show that this process depends critically on nanoscale fullerene crystallinity. It is expected that this conclusion applies more generally to the donor as well as other acceptors (nanocrystallinity of both D and A is not required), although this will depend on the degree of intermolecular electronic coupling within the crystallites, the strength of which may be one reason for the unique success of fullerenes as organic photovoltaic acceptors. Looking forward, it is important for theoretical efforts to include many molecules in modelling a DA HJ to accurately capture the role of transient extended states in the photogeneration process and support the design of new donor and acceptor material combinations with lower energy loss and higher open-circuit voltage. Device fabrication BHJ devices were fabricated by thermal evaporation onto pre-patterned indium tin oxide (ITO) contacts according to the structure: glass/ITO (100 nm)/MoO 3 (5 nm)/NPD:C 60 (40 nm)/bathocuproine (10 nm)/Ag (100 nm). The active layer composition was varied from 20 to 90% C 60 according to the relative co-deposition rates of NPD to C 60 in the ratios 4:1, 2:1, 1:1, 1:4 and 1:9. Films for PL were deposited separately on quartz followed by a 100-nm Ag layer to minimize substrate autofluorescence and maintain a comparable optical environment as in the electrical devices. All devices and films were packaged in a glove box using ultraviolet-curable epoxy and a glass cover to avoid atmospheric degradation. Device performance metrics measured under AM1.5G simulated 1 sun illumination are summarized in Supplementary Fig. 6 . Ellipsometry and X-ray diffraction Spectroscopic measurements on Si/SiO 2 (100 nm)/organic (NPD, C 60 or NPD:C 60 ; 50 nm) layers were conducted using a variable angle spectroscopic ellipsometer (Ges5, Sopralab); ellipsometry refractive index dispersions are shown in Supplementary Fig. 7 . On the same films, glancing incidence X-ray diffraction measurements were performed on a PANalytical X’Pert Pro Materials Research Diffractometer (PANalytical) using Cu Kα radiation. An integration time of 5 s per 2 θ of 0.01° was used for scanning 2 θ , with a fixed incident angle of 0.2°. Luminescence and EA EQE data were obtained using a standard monochromator and lock-in amplifier setup with a laser-driven Xe lamp source and a chopping frequency of 500 Hz. IQE was calculated from the balance of reflected and transmitted light measured in the same experiment (that is, IQE=EQE/(1− R − T )). EA data were acquired using the same system with light incident at an angle of ~15° through the ITO contact and collected in reflection from the Ag cathode (that is, a double pass in transmission through the active layer) using a Si photodiode. The devices were depleted at −1 V reverse bias and a 300 mVrms, f =1 kHz sinusoidal dither was applied to measure the rms change in transmitted light intensity. The linear absorption data in Fig. 5a of the text were collected in transmission differentially between two films with differing thickness (50 nm test film with a 10-nm reference film) in order to minimize the influence of reflection. Steady-state EL spectra were collected under direct current bias and PL spectra with 10 mW, λ =532 nm excitation using a fibre-coupled spectrograph with a cooled Si CCD array. Spectrally resolved PL transient data were obtained using a Hamamatsu C5680 streak camera and ~150 fs, 10 μJ cm −2 pump pulses at a pump wavelength of 530 nm and a repetition rate of 2 kHz. The transient spectra provided in Supplementary Fig. 8 confirm that the observed decay is due to emission from the CT state. The intensity of all spectra was calibrated using an Ocean Optics tungsten-halogen calibration lamp and is plotted in units proportional to photon flux/area/time/eV. Appropriate, non-fluorescing longpass filtres were employed in all measurements to avoid interference from grating doubles. Error bars for the EL and PL emission energies extracted via multipeak fitting reflect uncertainty to ±1 s.d. according to standard nonlinear regression analysis. Error bars associated with dielectric constant, EQE and device performance metrics in the Supplementary Information reflect ±1 s . d . in the result of measurements on multiple different devices with sample sizes ranging from 5 to 10. How to cite this article: Bernardo, B. et al. Delocalization and dielectric screening of charge transfer states in organic photovoltaic cells. Nat. Commun. 5:3245 doi: 10.1038/ncomms4245 (2014).